Undesired usage and the robust self-assembly of heterogeneous structures Inspired by multiprotein complexes in biology and recent successes in synthetic DNA tile and colloidal self-assembly, we study the spontaneous assembly of structures made of many kinds of components. The major challenge with achieving high assembly yield is eliminating incomplete or incorrectly bound structures. Here, we find that such undesired structures rapidly degrade yield with increasing structural size and complexity in diverse models of assembly, if component concentrations reflect the composition (that is, stoichiometry) of the desired structure. But this yield catastrophe can be mitigated by using highly non-stoichiometric concentrations. Our results support a general principle of ‘undesired usage’—concentrations of components should be chosen to account for how they are ‘used’ by undesired structures and not just by the desired structure. This principle could improve synthetic assembly methods, but also raises new questions about expression levels of proteins that form biological complexes such as the ribosome. A central feature of living systems is that they self-assemble their parts. Within the cell, an enormous variety of macromolecular complexes form spontaneously [1] , with nearly every part having different shape and binding affinities. These complexes range from structures with a small number of different components (chaperones and proteasomes) to large structures with complex topologies (the nuclear pore complex and the ribosome). Although the assembly pathways of such complexes have been investigated [2] , [3] , [4] , [5] , general design principles for binding energies, concentrations and other parameters of the self-assembly process are still mysterious. To minimize waste or errors, these complexes presumably assemble with high yield. Material synthesis strategies have also recently started to use large numbers of different components, particularly with nanostructures either coated [6] with or entirely composed of DNA [7] , [8] , [9] , [10] . For example, work [7] , [8] , [11] , [12] , [13] on assemblies of short DNA strands has now been extended to a plethora of complex large shapes called tile or ‘brick’ [9] , [10] assemblies. Similar efforts are underway using rationally designed proteins [14] , [15] or colloidal particles [16] with specific interactions. The major challenge with achieving high yield is eliminating competing undesired structures. Even when components are chosen so that the desired structure is the ground state, incomplete and incorrectly formed structures will occur. Incomplete structures can result from a lack of sufficient components to drive the reaction to completion. Incorrectly bound structures can result from inevitable nonspecific binding between components. Such crosstalking interactions are ubiquitous in both natural and synthetic systems. Nonspecific interactions between proteins arise from protein structure constraints [17] , [18] , creating challenges for both signalling pathways [19] and self-assembly [12] , [20] . In DNA brick assembly [9] , [10] , even with designer DNA sequences that precisely match the desired structure, there is still (weaker) binding affinity of each strand to other general components. The number of undesired structures of varying size and composition grows exponentially with the number of component types in the desired structure [21] , [22] , [23] , [24] , [25] . A fundamental question is whether undesired structures can be sufficiently suppressed by choosing the binding energies [26] , [27] and concentrations [28] of different components. Within biology, it is believed that the concentrations of individual proteins of multiprotein complexes obey the dosage balance hypothesis (DBH) [29] , which asserts that the optimal expression levels are proportional to the stoichiometric ratio in which proteins form complexes. Likewise, the synthetic examples that we are aware of choose concentrations of individual components to match the stoichiometry of the desired structure. However, there is no evidence that stoichiometrically balanced concentrations maximize assembly yield. We study these questions in a broad set of models relevant to protein complexes, DNA brick and colloidal assemblies. Individual structures are represented by their connectivity graphs ( Fig. 1 ), which we then model with multivalent components with short ranged binding affinity. Our models build upon a framework introduced [12] , [13] , [30] in the context of DNA tiles. 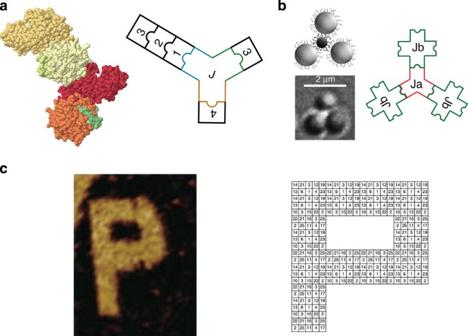Figure 1: Abstraction of multiprotein complexes, colloidal structures and DNA ‘brick’ assemblies. (a) The protein complex is a platelet-receptor complex involving thrombin, necessary for platelet aggregation56(classified by topology in ref.1). (b) The colloidal structure is made of two kinds of DNA-coated particles38with valence imposed through geometry, whereas (c) the P-shaped structure is made of dozens of DNA strands called ‘bricks’9. We model assembly using multiple component species with independent concentrations and demonstrate their role in suppressing undesired structures. Image permissions: reprinted (adapted) by permission from (a) RCSB PDB (http://www.rcsb.org) of PDB ID 1P8V (ref.56). (b)The American Physical Society38, copyright 2013, (c) Macmillan Publishers Ltd9, copyright 2012. Figure 1: Abstraction of multiprotein complexes, colloidal structures and DNA ‘brick’ assemblies. ( a ) The protein complex is a platelet-receptor complex involving thrombin, necessary for platelet aggregation [56] (classified by topology in ref. 1 ). ( b ) The colloidal structure is made of two kinds of DNA-coated particles [38] with valence imposed through geometry, whereas ( c ) the P-shaped structure is made of dozens of DNA strands called ‘bricks’ [9] . We model assembly using multiple component species with independent concentrations and demonstrate their role in suppressing undesired structures. Image permissions: reprinted (adapted) by permission from ( a ) RCSB PDB ( http://www.rcsb.org ) of PDB ID 1P8V (ref. 56 ). ( b )The American Physical Society [38] , copyright 2013, ( c ) Macmillan Publishers Ltd [9] , copyright 2012. Full size image Our analysis of these models suggests a simple new principle of ‘undesired usage’: control parameters such as component concentrations should be chosen based on how those components are ‘used’ by undesired structures, as opposed to just the desired structure. For example, if undesired structures ‘use’ component A more often than component B, A should be supplied in smaller amounts than B—even if the desired structure is made of one A and one B. We give a mathematical definition of ‘usage’ and show that this principle leads to regimes with markedly higher yields in diverse models of assembly, relevant to protein complexes, DNA-based self-assembly and colloidal assemblies. We first rigorously establish these results in an equilibrium model of self-assembly, introducing a perturbative Feynman diagram technique for computing yield that accounts for the combinatorial explosion of competing structures. We then demonstrate that the principle of undesired usage can also alleviate kinetic yield catastrophes in non-equilibrium models, focusing on two models of recent interest in colloidal and DNA brick assembly. In the systems we study, the yield improvement from non-stoichiometric concentrations is typically larger when the stoichiometric concentrations yield is smaller. Undesired usage must balance desired usage We consider self-assembly of heterogeneous structures made of n components; each component is one of m species types and has multiple distinct binding sites. Besides the desired structure, the m species of components can assemble numerous incomplete or incorrect undesired structures. (See Fig. 2 where m = n =4.) Incomplete structures are pieces of the desired structure that do not have all the necessary components, whereas incorrectly bound structures contain weak ‘crosstalking’ interactions. Such undesired structures vary in size, shape and composition and can markedly reduce yield. 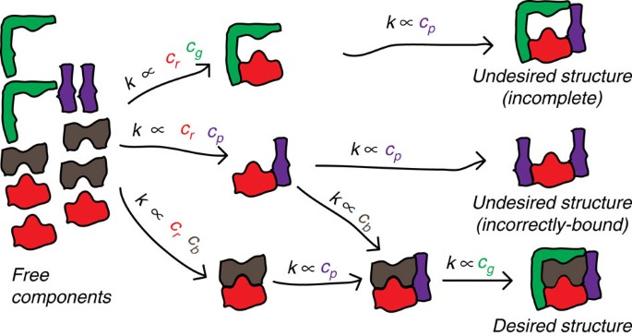Figure 2: Kinetic pathways leading to desired and undesired structures. Effective rate constantsk(and hence fluxes) along different pathways depend on concentrationsciof species in differing ways. Yield is improved by decreasing concentrations of species with high ‘undesired usage’, that is, species that increase flux along undesired pathways. Hence, optimal concentrationscimay differ greatly from the stoichiometry of the desired structure. For the schematic selection of pathways shown here, yield might be improved if concentrationcbis higher thancp,cgas lowcpandcgsuppress incorrect and incomplete structures, respectively. Figure 2: Kinetic pathways leading to desired and undesired structures. Effective rate constants k (and hence fluxes) along different pathways depend on concentrations c i of species in differing ways. Yield is improved by decreasing concentrations of species with high ‘undesired usage’, that is, species that increase flux along undesired pathways. Hence, optimal concentrations c i may differ greatly from the stoichiometry of the desired structure. For the schematic selection of pathways shown here, yield might be improved if concentration c b is higher than c p , c g as low c p and c g suppress incorrect and incomplete structures, respectively. Full size image We define yield Y as the number of desired structures produced relative to all undesired structures. That is, where X d ( c i ), X u ( c i ) are the numbers of desired and undesired structures produced by assembly and which depend on species concentrations c i . X u can be written as a sum over all undesired structures a , . We define the ‘usage’ of species i by structure a: reflects how the production rate of structure a depends on the concentration of component i . For example, consider an experiment carried out using concentrations c i and then perturb around these concentrations, c i → f i c i . If the perturbations are small, we can Taylor expand to write . Thus, large usage implies that increasing the concentration of species i will greatly increase the production of structure a. The gradient of yield with respect to log c i can be written in terms of usage, where the average is over all undesired structures a, each weighted by the amount X a of it produced. The proportionality constant in equation (3) is always positive. This equation defines the principle of undesired usage—yield is improved by lowering the concentration of component i whose average undesired usage is higher than its correct usage (and vice-versa). Changing concentrations in such a manner produces different distributions of undesired structures X a / X u , whose average undesired usage is closer to the correct usage . The resulting optimal concentrations can be very different from the stoichiometry in the desired structure. Our analysis of specific models will show that the resulting yield improvements are marked. In what follows, we apply this principle to equilibrium assembly as well as to two paradigmatic kinetic examples. In our model of equilibrium assembly, c i and X a in equation (2) will refer to steady-state concentrations, and we analytically show that the usage is the number of occurrences of species i in structure a. In our kinetic models, quantifies the dependence of the final amount X a of structure a on initial concentrations c i that deplete with time. Thus, equation (3) can be applied to both steady-state or initial concentrations and to equilibrium or kinetic assembly. Equilibrium assembly and yield catastrophes We begin by studying equilibrium assembly. We assume that the interactions between binding sites in the desired structure are strong and of energy s k B T <0. For example, in Fig. 3 , components 6 and 7 and components 4 and J 1 have strong binding with each other. In many systems, such as DNA bricks designed with random sequences or protein assemblies, the strong interaction energy will typically vary across the structure. Optimal concentrations will depend on such variation in binding energies and can be computed using the framework we introduce below; for simplicity, we focus on the case of a single strong binding energy scale s k B T and discuss generalizations in Supplementary Note 1 . 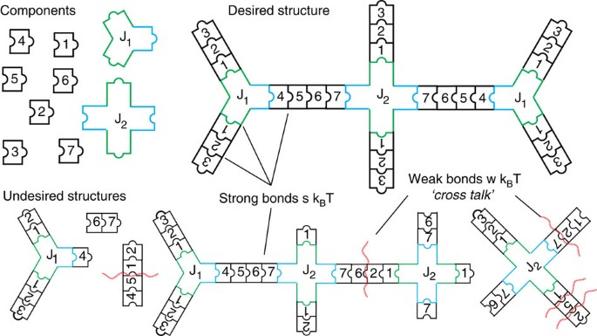Figure 3: Crosstalk leads to an exponential number of undesired competing structures. In our model of equilibrium assembly, desired structures of sizenare built frommspecies of bivalent and multivalent components, supplied at chemical potentialsμ1,μ2,…,μm. (n=29,m=9 here.) All bonds present in the millipede-like desired structure are strong (energys<0). All other bonds correspond to weak ‘crosstalk’ interactions (wavy red lines, energyw<0). Undesired structures made of weak bonds are energetically suppressed by factors ofe−β(w−s), but the number of such structures is exponentially large inn. Yield is determined by this energy–entropy balance. Figure 3: Crosstalk leads to an exponential number of undesired competing structures. In our model of equilibrium assembly, desired structures of size n are built from m species of bivalent and multivalent components, supplied at chemical potentials μ 1 , μ 2 ,…, μ m . ( n =29, m =9 here.) All bonds present in the millipede-like desired structure are strong (energy s <0). All other bonds correspond to weak ‘crosstalk’ interactions (wavy red lines, energy w <0). Undesired structures made of weak bonds are energetically suppressed by factors of e − β ( w − s ) , but the number of such structures is exponentially large in n . Yield is determined by this energy–entropy balance. Full size image In any natural or synthetic system, there is always some level of nonspecific interactions that we call ‘crosstalk’ [12] , [18] , [20] , [31] , [32] , [33] . To model crosstalk, we assume that all non-desired binding sites interact weakly with an energy w k B T <0 that is distributed randomly as ρ ( w ). Thus, components 6 and 2 interact through such a weak crosstalk interaction. The ‘male’ site of component 3 interacts weakly with all components since it is unbound in the desired structure. We assume for now that each component i is supplied at a fixed chemical potential μ i , so the concentration of free components has the constant value , with . This steady-state model mimics the assembly of the ribosome and other macromolecular complexes whose protein components are being continually produced, or assembly in a large sea of components whose concentrations change very little during assembly. Recent works [10] , [34] , [35] suggest that, in some temperature regimes, the experiments of [9] , [10] can be described in such a manner. See kinetic models below for complementary possibilities. Yield at equilibrium can be obtained by summing the partition function over all undesired structures; we developed a method adapted from Feynman diagrams to perform such numerical computations efficiently (see Methods section). We find that yield is determined by an energy–entropy balance, with the number of the most stable competing structures growing as ~ n 2 and each such crosstalk-containing structure suppressed by an energetic factor of e − β ( w − s ) . Building structures of size n with any yield at all requires the energetic suppression to dominate which in turn implies a bound on the crosstalk energy w . Extending such analytic arguments (detailed in Supplementary Note 2 and Supplementary Fig. 5 ), we find , where is the exponential average of crosstalk energies w between all species, assumed to be distributed as ρ ( w ). A and B are O (1) numbers that depend on the topology of the desired structure. Note that stronger interactions correspond to more negative energies in our convention. If crosstalk strength w exceeds this bound, the different species of components are indistinguishable and the system effectively behaves as having only one species. Hence, we will restrict ourselves to crosstalk below this bound (which we call the ‘ crosstalk threshold’) and examine how the maximum yield depends on the size and structural complexity of the desired structures. Equal chemical potentials lead to a yield catastrophe. For simplicity, we begin by considering structures where all components are distinct, that is, the number m of distinct species used is also the size n of the structure. We first assume that the chemical potentials of all m = n species are stoichiometric, so μ i = μ . 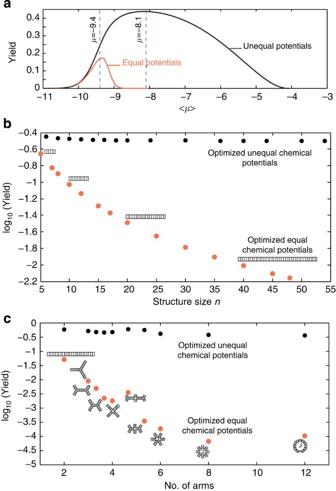Figure 4: Alleviation of the yield catastrophe. (a) Yield is maximized at an intermediate average chemical potential that favours neither large aggregates nor small incomplete structures. Yield is shown for a linear structure of sizen=m= 8 as a function of the average chemical potential. (b,c) Yield falls (red) with (b) size and (c) increasing number of arms if the chemical potentials of different components are equal. The yield improvement owing to optimized unequal potentials is greater for larger and highly branched structures. The resulting optimized yield (black) is relatively independent of shape and size. (n=mfor all structures. Ina,w=−2kBT,g=w−s=−10kBT. Inb, to compare differentnfairly, we scaledto keepw−sa constant amount over thecrosstalk threshold. All shapes inchaven=25, withg=12kBT,w=−2kBT.) Figure 4a shows the yield (red curve) as a function of μ , for a linear structure of size n =8. Low chemical potentials favour incomplete structures, whereas high potentials favour large aggregates held together by weak bonds; yield is maximized for an intermediate value of μ . Figure 4: Alleviation of the yield catastrophe. ( a ) Yield is maximized at an intermediate average chemical potential that favours neither large aggregates nor small incomplete structures. Yield is shown for a linear structure of size n = m = 8 as a function of the average chemical potential . ( b , c ) Yield falls (red) with ( b ) size and ( c ) increasing number of arms if the chemical potentials of different components are equal. The yield improvement owing to optimized unequal potentials is greater for larger and highly branched structures. The resulting optimized yield (black) is relatively independent of shape and size. ( n = m for all structures. In a , w =−2 k B T , g = w − s =−10 k B T . In b , to compare different n fairly, we scaled to keep w − s a constant amount over the crosstalk threshold. All shapes in c have n =25, with g =12 k B T , w =−2 k B T .) Full size image The red data points in Fig. 4b show how this maximum yield depends on n , the size of the linear structure. To fairly compare yields for structures of different n , we need to increase the difference g = w − s between strong and weak bond energies as , so that g stays above the crosstalk threshold by a fixed amount G . We set A =2.0 for linear structures. Strikingly, the yield degrades exponentially with increasing n , indicating that by n ≈35 the maximum yield is at most ~1%. The yield degrades because the number of competing structures increases markedly with increasing size n ; although each individual competing structure has higher energy, the combinatorial explosion of possibilities with growing n strongly limits the yield. This yield catastrophe also occurs with increasing structural complexity. Using the Feynman method, we numerically computed the yield of branched structures for fixed n , but with increasing numbers of arms ( Fig. 4c ). Again, we find that the yield decreases exponentially with the number of arms; the reason is that the number of competing structures increases markedly with the number of arms (calculated in Supplementary Note 1 ). The yield catastrophe presents a fundamental constraint: if the concentrations of components are stoichiometrically matched to the structure, then there is a limit to how large and how complex a structure can be robustly assembled. Unequal chemical potentials alleviate the yield catastrophe . We now allow the components to have unequal chemical potentials μ i . We numerically vary μ i independently to optimize yield, using gradient descent on our Feynman construction for partition functions. Strikingly, the optimal values of μ i are highly non-uniform across the structure, with exterior pieces having much higher μ i (and hence concentrations) than interior pieces. Moreover, the optimal μ i s lead to a nearly complete recovery from the yield catastrophe. Figure 4 shows the effect on our two model calculations: Fig. 4b,c (black dots) show that the optimal μ i s lead to a yield that is independent of the length n of linear structures and the number of arms a in branched structures. To understand why the optimal μ i s are unequal, we analyse undesired usage. In equilibrium, the ‘usage’ of species i by structure a, defined in equation (2), simply reduces to the number of times species i occurs in structure a (see derivation in Methods section). 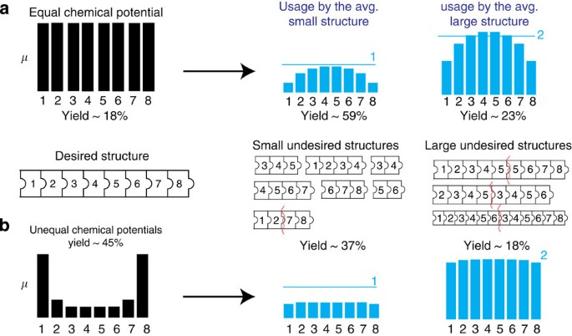Figure 5: Exploiting undesired usage. (a) Interior components have higher undesired usage than desired usage (and vice-versa for exterior components), when assembly is carried out with equal chemical potentials. For example, the undesired usage of5by large structures is higher (≈ 2) than its desired usage (=1). (b) Hence, as dictated by undesired usage (equation (3)), decreasingμ5and increasingμ1suppresses large and small structures relative to the desired structure, respectively. At the optimal U-shaped profile shown inb, the undesired usage of all components matches usage in the desired structure. Avg., average. Figure 5 shows the implications of usage graphically; we plot the undesired usage of components i = 1,…8 averaged over competing structures grouped as larger and smaller than the desired structure. With equal chemical potentials ( Fig. 5a ), only 60% of small undesired structures contain component 1 but almost 90% of them contain 5 . This asymmetry arises because, for example, the dominant small structures of length four are 1234 , 2345 , 3456 , 4567 , 5678 (others, such as 1278 , are suppressed by weak bonds). Component 5 occurs in most of these structures while 1 occurs in only one. Large structures have unequal usage for similar reasons. Figure 5: Exploiting undesired usage. ( a ) Interior components have higher undesired usage than desired usage (and vice-versa for exterior components), when assembly is carried out with equal chemical potentials. For example, the undesired usage of 5 by large structures is higher (≈ 2) than its desired usage (=1). ( b ) Hence, as dictated by undesired usage (equation (3)), decreasing μ 5 and increasing μ 1 suppresses large and small structures relative to the desired structure, respectively. At the optimal U-shaped profile shown in b , the undesired usage of all components matches usage in the desired structure. Avg., average. Full size image In the desired structure, each component is only used once. Hence, increasing the supply of 1 (that is, increasing μ 1 ) will suppress small structures (whose usage of 1 is 0.6) relative to the desired structure while only somewhat enhancing large structures (whose usage of 1 is 1.1). The suppression of small structures dominates and yield is improved. Similarly, decreasing μ 5 will improve yield by greatly suppressing large structures (usage ≈2) and somewhat enhancing small structures (usage ≈0.9). Modifying chemical potentials in this way changes the distribution of competing structures produced and hence usage will have to be recomputed. The process terminates when the undesired usage of different components matches the stoichiometry in the desired structure (see equation (3) and Fig. 5b ). Increasing μ 1 any further will promote large structures more than it suppresses small structures. Similarly decreasing μ 5 any further will promote small structures and harm yield. In this way, the optimal supply of components strikes a balance between different groups of competing structures. Undesired usage analysis also explains the optimal profiles for general branched structures shown in Fig. 6 ; for example, the dominant competing structures for the 3-armed star in Fig. 6a consist of junction J with partially built arms. These partial arms will almost always contain component 1 and not contain component 3 unless it is a complete arm. Partial arms in which component 3 occurs without 1 involve crosstalking interactions and contribute less to the partition function. In the millipede-like structure, junction J 2 is to have lower concentration than J 1 , since J 2 , with four sites, is more prone to self-aggregation. See Supplementary Figs 1–3 and Supplementary Note 1 for a sampling of such competing structures, further usage analysis of structures shown here and the weak dependence of optimized yield on topology of structures in Fig. 4c . 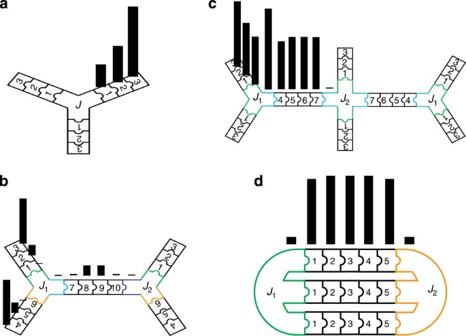Figure 6: Optimal chemical potential profiles. Highly non-stoichiometric potentials optimize yield for (a) a star, (b) an H, (c) a millipede-like and (d) a double-looped Θ-like structure; for example,ina. Yield improvement over using equal potentials (with the same average concentration of free components) is ≈ 2 × , ≈ 36 × , 2,800 × and 1.8 × for the star, H, millipede and Θ structures, respectively. (Numeric details inSupplementary Note 1.) Figure 6: Optimal chemical potential profiles. Highly non-stoichiometric potentials optimize yield for ( a ) a star, ( b ) an H, ( c ) a millipede-like and ( d ) a double-looped Θ-like structure; for example, in a . Yield improvement over using equal potentials (with the same average concentration of free components) is ≈ 2 × , ≈ 36 × , 2,800 × and 1.8 × for the star, H, millipede and Θ structures, respectively. (Numeric details in Supplementary Note 1 .) Full size image In Supplementary Fig. 4 , we show how the optimal concentration profile changes if the strong binding energy s varies across the structure; we show that our results on the yield catastrophe and its alleviation continue to hold. In summary, we see marked yield improvement ( Fig. 4 ) by using unequal chemical potentials as dictated by undesired usage (equation (3)). Thus, unequal potentials provide sufficient ‘control knobs’ to suppress competing structures whose number is exponential in size n . Undesired usage analysis alleviates kinetic yield catastrophes Thus far, we have analysed the mitigation of the equilibrium yield catastrophe using the principle of undesired usage. However, assembly in many systems is limited by kinetics. Unlike equilibrium yield, the details of kinetic pathways differ from system to system. Nonetheless, equation (3) shows that undesired usage analysis still applies, although the definition of usage depends on the details of the kinetics. Here we examine complementary exemplars of kinetic issues in models of two synthetic systems—DNA brick and irreversible colloidal assemblies. In both cases, we show that non-stoichiometric concentrations markedly alleviate yield catastrophes. In the kinetic problems we study here, concentrations c i will refer to the initial amounts of components supplied, since free components are significantly depleted over the course of assembly. Incomplete incompatible structures . Kinetic yield catastrophes can occur even in the absence of crosstalk. Our first model assumes that a desired structure can nucleate and grow from several inequivalent seeds ( Fig. 7a ). If the rate of nucleation is comparable or fast compared with the rate of subsequent growth of seeds into full structures, many inequivalent seeds will nucleate and grow in parallel. Such parallel growth can lead to a kinetic yield catastrophe in the form of a ‘depletion trap’; all components are locked up in incomplete incompatible structures. 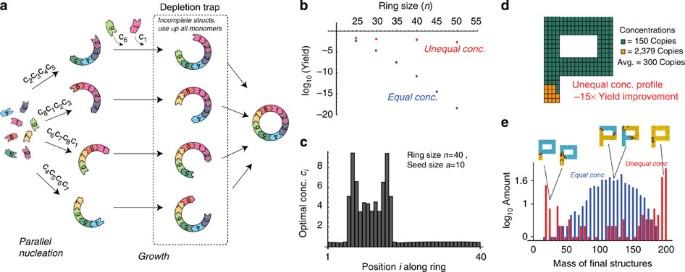Figure 7: Non-stoichiometric concentrations can avoid depletion traps created by rapid parallel nucleation of distinct seeds. (a) If nucleation is faster than subsequent growth into full rings, all free components can be locked up in the set of incomplete structures shown in the dotted box. These structures cannot grow further since they lack free components and the ability to bind each other. (b) Depletion traps are more severe for larger structure sizesn, resulting in a kinetic yield catastrophe; yield with equal concentrations falls exponentially withn(blue dots). (c) The unequal concentrations shown forn=40 selectively choose one nucleation path inaover others. Hence, the depletion trap is mitigated and yield improvement is marked (red dots inb). (d) Yield of a 2-dimP-structure made of 208 distinct species of tiles, resembling DNA brick assemblies9, is also improved by unequal concentrations. (e) With equal concentrations, a depletion trap results in incomplete structures of typical size ~100–150 (blue bars). With the unequal profile ind, the depletion trap is resolved; final structures are either of full size 208 or remain small seeds of size ~20 (red bars). Figure 7: Non-stoichiometric concentrations can avoid depletion traps created by rapid parallel nucleation of distinct seeds. ( a ) If nucleation is faster than subsequent growth into full rings, all free components can be locked up in the set of incomplete structures shown in the dotted box. These structures cannot grow further since they lack free components and the ability to bind each other. ( b ) Depletion traps are more severe for larger structure sizes n , resulting in a kinetic yield catastrophe; yield with equal concentrations falls exponentially with n (blue dots). ( c ) The unequal concentrations shown for n =40 selectively choose one nucleation path in a over others. Hence, the depletion trap is mitigated and yield improvement is marked (red dots in b ). ( d ) Yield of a 2-dim P -structure made of 208 distinct species of tiles, resembling DNA brick assemblies [9] , is also improved by unequal concentrations. ( e ) With equal concentrations, a depletion trap results in incomplete structures of typical size ~100–150 (blue bars). With the unequal profile in d , the depletion trap is resolved; final structures are either of full size 208 or remain small seeds of size ~20 (red bars). Full size image The problem of incomplete structures has been argued to be central to both DNA brick assembly [9] , [34] , [35] , [36] and protein complexes [27] , [37] . Indeed, before the experiments of ref. 9 , such depletion traps were thought to make DNA brick-like approaches unlikely to succeed. Recent simulations [34] show that in a narrow regime of parameter space, assembly is successful because nucleation is sufficiently slow compared with growth, that is, each nucleated structure typically completes growth before the nucleation of another seed. However, outside of this regime, multiple structures nucleate rapidly, deplete monomers and might incorrectly bind each other [34] . Hence, it is important to develop strategies that expand the range of conditions for successful assembly; other materials, assembly conditions and larger target structures may not satisfy the criterion of slow nucleation and fast growth. Undesired usage analysis implies that unequal concentrations can alleviate depletion traps. We first demonstrate this in a simple nucleation-and-growth model of a ring ( Fig. 7a ), where the ring is made of n bivalent components that bind only to their correct partners. We assume that the interactions are cooperative (for example, through allostery) so that the ring grows from critical nucleating seeds of size a or greater: structures smaller than size a quickly dissolve into monomers, but a nucleating seed of size a grows irreversibly [30] . Assembly starts with an initial supply of components of concentration c i , i =1,…, n that is depleted over time. We compute yield by numerically solving the master equation with initial conditions c i (see Methods section). With equal concentrations, we find that the depletion trap strongly degrades yield for large n ; this degradation occurs because the nucleation rate of seeds is independent of structure size n while the subsequent growth rate of the seed into the full structure falls as 1/ n . Further, the number of parallel nucleation pathways increases as n . Hence, yield falls exponentially with increasing structure size n , giving a kinetic yield catastrophe ( Fig. 7b ). With unequal concentrations, this depletion trap is strongly alleviated. Through gradient descent optimization, we find that the optimal concentration profile is highly non-uniform ( Fig. 7c ), with high concentrations for a region of size ~ a and low concentrations everywhere else. (By symmetry, this high concentration region can be anywhere around the ring.) The unequal concentrations greatly enhance nucleation for one of the many assembly parallel paths shown in Fig. 7a , suppressing the rest. Hence, even with slow growth, the components needed for growth are not significantly depleted by competing pathways, with a marked effect on yield (red dots in Fig. 7b ). We validated these same conclusions in a 2-dim ‘P’-shaped structure ( Fig. 7d ), made of n =208 tiles and resembling DNA brick assemblies [9] . We assume that each tile in the structure is a unique species with four distinct binding sites that bind only to their correct partners. We simulated a nucleation-and-growth model similar to the ring above (see Methods section); seeds of size a =18 could nucleate anywhere in the structure and then grow irreversibly, with the rates of both processes determined by the concentrations of components. Starting assembly with equal amounts (300 copies) of each species, we find a severe depletion trap, resulting in a wide distribution of incomplete structures of typical size ~100–150 tiles (blue bars in Fig. 7e ). Only nine structures are of size within 15% of the complete n =208 P-structure. On the other hand, the highly unequal profile (with the same average number 300 as earlier) shown as a heatmap in Fig. 7d , gives a yield of ~135 structures, a 15-fold improvement. Incomplete sticky structures . Colloidal particles form aggregates easily because they are isotropically sticky and pick up multiple partners, making it difficult to build predictable finite structures. Such a yield catastrophe was recently observed [38] and mitigated using highly non-stoichiometric concentrations. Finite clusters of type AB 4 were built from two kinds of DNA-coated colloidal particles A and B, designed so as to bind each other irreversibly but not bind their own kind. The radii of A and B were chosen so that exactly four Bs bind to each A. 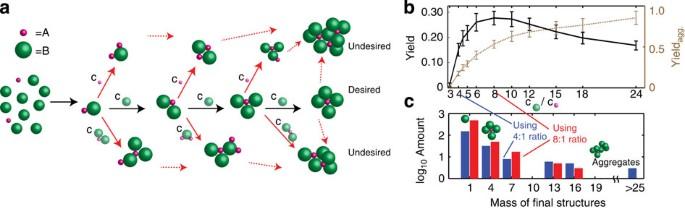Figure 8: Non-stoichiometric concentrations can suppress undesired aggregation in irreversible colloidal assembly. (a) In the experiments of38, incomplete structures can incorrectly glue to each other (red arrows), greatly reducing yield. However, red pathways leading to undesired aggregates (agg.) have higher usage of particle A than the black pathway leading to the desired AB4structure. Hence, a high ratio of initial concentrationscB/cAmarkedly increases yield; incomplete structures are rapidly completed by B particles along the black path, with low probability of taking any red branches. (b) Using a stochastic simulation of these pathways, we find that yield peaks atcB:cA= 8:1. (c) IfcB:cA= 4:1 (stoichiometric ratio) instead, the distribution of assembled structures is shifted towards larger aggregates (blue bars) and hence yield is lower. Inb, we also plot an alternative notion of yield, yieldagg., relevant to the experiments in ref.38, which considers only large aggregates as undesirable and disregards excess A or B particles, which are easily washed out. Yieldagg.increases indefinitely withcB/cA. Figure 8a shows a selection of kinetic pathways leading to the desired AB 4 structure (black) and to several undesired aggregates (red). The main hurdle to high assembly yield is ensuring that incomplete structures (that is, AB, AB 2 and AB 3 ) bind only to particle B and not to other incomplete structures, A, or larger aggregates. The experiments [38] found large aggregates and a very low yield of AB 4 if assembly starts with the stoichiometric ratio 4:1 of B:A. On the other hand, supplying a large excess of B greatly enhanced the yield of AB 4 . Figure 8: Non-stoichiometric concentrations can suppress undesired aggregation in irreversible colloidal assembly. ( a ) In the experiments of [38] , incomplete structures can incorrectly glue to each other (red arrows), greatly reducing yield. However, red pathways leading to undesired aggregates (agg.) have higher usage of particle A than the black pathway leading to the desired AB 4 structure. Hence, a high ratio of initial concentrations c B / c A markedly increases yield; incomplete structures are rapidly completed by B particles along the black path, with low probability of taking any red branches. ( b ) Using a stochastic simulation of these pathways, we find that yield peaks at c B : c A = 8:1. ( c ) If c B : c A = 4:1 (stoichiometric ratio) instead, the distribution of assembled structures is shifted towards larger aggregates (blue bars) and hence yield is lower. In b , we also plot an alternative notion of yield, yield agg. , relevant to the experiments in ref. 38 , which considers only large aggregates as undesirable and disregards excess A or B particles, which are easily washed out. Yield agg. increases indefinitely with c B / c A . Full size image We were able to reproduce this behaviour with the stochastic simulation of a simple model of irreversible aggregation (see Methods section). Yield is maximized at the highly non-stoichiometric ratio of 8:1 for B:A ( Fig. 8b ). Figure 8c (red bars) shows that the 8:1 supply shifts the distribution of assembled structures towards lower mass, compared with a 4:1 supply (blue bars). An excess of B suppresses the probability of taking the red pathways, relative to the correct black pathway ( Fig. 8a ). The depletion of free A particles with time helps further suppress undesired pathways—otherwise, the desired structure AB 4 can pick up free As and aggregate. Hence, a high ratio of B:A helps rapidly complete incomplete structures through addition of monomers and prevent them from sticking to each other. The results here generalize Flory's classic theory of irreversible condensation [39] that involved only a small number of species. These complementary examples from DNA, protein and colloidal assembly demonstrate that undesired usage analysis can greatly enhance yield in examples where assembly is kinetically controlled. Unlike our equilibrium examples, the character of kinetic yield catastrophes depends on modelling assumptions; for example, numerical prefactors in nucleation and growth rates, reversibility of growth and so on, which vary across different systems. Nevertheless, using unequal concentrations markedly alleviates kinetic yield catastrophes, especially when kinetic traps are strong. We leave a study of unequal concentrations using kinetic models tailored to particular systems such as colloids or DNA brick assemblies (for example, along the lines of refs 25 , 34 ) to future work. We have studied strategies to suppress undesired structures that can catastrophically reduce the assembly yield of complex heterogeneous structures. The central lesson of our work is that the supply of different components should account for their ‘usage’ by undesired structures. The resulting optimal concentrations can differ greatly from the stoichiometry of the desired structure itself. We have shown that undesired usage analysis is a useful consideration to apply to a range of assembly experiments involving DNA, colloids and proteins [9] , [10] , [14] , [15] , [40] , in both equilibrium and highly kinetic conditions, even if the precise degree of kinetic yield improvement is hard to predict without knowledge of the detailed kinetics. We leave the extensions to more complex kinetic models [41] , [42] , [43] such as hierarchical assembly to future work. Our framework and results have precedence in earlier work on the impact of concentrations in specific models of micelles [44] , polymer condensation [39] and protein complexes [37] . Chen and Kao [28] studied a DNA tile model with crosstalk and found that optimal concentrations are proportional to the square root of stoichiometric ratios. They assume that correct bonds are irreversible. In contrast, we used a fully reversible crosstalk model that describes intrinsically more error-prone assembly and showed that even catastrophically low yields can be restored by non-stoichiometric concentrations. As a result, while our results are similar in spirit, yield improvements found in ref. 28 are weaker than those reported here. Our results also differ because our physical partition function treatment accounts for all possible erroneous structures while ref. 28 used a heuristic local definition of errors. The principle of undesired usage can be generalized to other control parameters beyond concentrations. For example, unequal binding energies are expected to alleviate yield catastrophes in our linearly branched models and in depletion trap models [27] . These results differ from earlier analyses [26] that only considered competing structures of the same size as the desired structure (that is, not bulk assembly). The design of structure itself [45] can be subject to undesired usage analysis; given a physical structure, how should it be composed of different species to minimize assembly of competing structures? Finally, in practice, some structures might be more undesirable than others, owing to their being more difficult to separate or more toxic in a cell. Our framework can be generalized to accommodate such varying functional costs ( Supplementary Note 4 ), providing a way to produce the least undesirable mix of structures appropriate in a given functional context. Biology has many examples of heterogeneous multiprotein/RNA complexes [1] , ranging from simple linear complexes to ribosomes and the nuclear pore complex. Our work predicts that optimal expression levels of components of large protein complexes can be highly non-uniform; for example, if a protein component is particularly likely to form toxic aggregates, that protein should be expressed at lower levels than other complex components. Phrased this way, the implications of our work seem intuitive and perhaps even obvious—and yet they seemingly contradict a common formulation of the DBH [29] , [46] , [47] , [48] . DBH states that the optimal expression levels for complex-forming proteins is stoichiometric and that deviations have large fitness costs. Such fitness costs are believed to be a strong evolutionary constraint on gene duplication events, aneuploidy, gene family sizes and dominance. Instead, our results suggest that the optimal expression level baseline may differ greatly from stoichiometry due to undesired structures. However, the rest of DBH—that changes from this optimal level have large fitness costs—would still apply about this modified baseline. We note that all the strong evidence for DBH involves changes in expression levels [29] , [46] ; such evidence includes experiments that enhance or repress expression of select proteins and statistical studies of gene duplication events. These data say little about what the optimal ratios are in the first place. In fact, the database consensus for expression levels of proteins involved in complexes is highly uneven across those complexes (ref. 49 and Supplementary Note 4 and Supplementary Fig. 6 ). Our proposal also finds support in the work of refs 20 , 31 , which found that highly promiscuous proteins in yeast have lower expression levels. The production of proteins comes at a cost (energy, material and time) to the cell and highly unequal production of proteins needed in equal amounts seems wasteful, unless some other benefit were conferred [49] , [50] . However, expression levels need to be measured more accurately to draw further conclusions. Finally, it is intriguing to ask how the organization of operons—sets of bacterial genes whose expression is regulated together—is related to potential undesired complexes [51] , [52] . There is evidence for such connections between genome structure and the physics of protein complexes in other contexts [53] , [54] . We leave a detailed study of these questions to future work. Equilibrium assembly and Feynman expansion Our model has m species of multivalent particles with distinguishable binding sites as shown in Fig. 3 . The desired structure defines the interaction energy between pairs of binding sites on two different particles. If a pair of sites is bound in the desired structure, the binding is strong and of energy sk B T ; else, the binding energy is wk B T (a weak ‘crosstalk’ interaction). Each species is supplied at a steady chemical potential μ i (or equivalently concentration where . We define g = w − s . At equilibrium, yield can be written in terms of partition functions of desired and undesired structures; in equation (1), X d = Z d and where Z a is the partition function of structure a, where p is the total number of bonds in a , q is the number of crosstalking bonds and g = w − s >0 is the difference between the strong and weak bond energies. is the sum of chemical potentials over all particles k (of species type i k ) present in structure a. Since X a = Z a at equilibrium and , equation (4) implies that usage at equilibrium is simply given by the number of occurrences of species i in structure a. Feynman method Finding the yield requires summing the partition function over all competing structures a of varying shapes and sizes as shown in Fig. 3 ; the list can be quite large even for a simple structure. We markedly simplified such tedious calculations by developing a perturbative method for computing the partition functions of linearly branched and/or looped structures based on rules adapted from Feynman diagrams. Feynman methods have been used before in the computation of partition functions of polymers [55] . In our context, Feynman rules give us a one-step method of summing over structures of all sizes that are consistent with a given topology. The Feynman rules here are: (1) A linear segment made of any number of bivalent components between two junctions is associated with the matrix D i j . where E ij is the interaction energy between species i and j , binding in the order i − j , and c j are the concentrations of components. (2) Every binding site p of a junction J is associated with a row vector (column vector if site p is female) where E pi is the binding energy of p to bivalent species i . In addition, each junction J is associated with a concentration factor c J . 3. Free ends of linear segments are associated with a special vector that can account for solvent–component interactions. We take in this paper. To find the partition function summed over all structures with a given topology, we first carry out matrix multiplication of the row and column vectors associated with junctions (or free ends) and the matrix D i j associated with the linear segment between such junctions, giving a scalar factor of the type . The total partition function is the product of all such scalar factors associated with a given topology. The Feynman method is particularly efficient when the number of bivalent species is large, as long as the number of species with valence larger than two stays small. Supplementary Fig. 1 and Supplementary Note 1 contain detailed derivations and examples of applying these Feynman rules. Kinetic depletion trap Ring . The ring structure is modelled as made of n bivalent particles, each of a distinct species. The left binding site on species i −1 will bind only to the right binding site of i ; for example, in Fig. 7a , the left site of species 5 will only bind the right site of 6. Correct binding is irreversible and no incorrect binding is allowed. Particle n is assumed to bind to 1, allowing assembly of a ring. We denote concentration of species i by positive real numbers C i ( t ), i = 1… n . The concentration of a clockwise segment of the ring from i to j is denoted X ij ( t ); we assume modular (mod n ) arithmetic for indices. Structures of size less than a critical nucleation size a are assumed to quickly dissolve back into monomers. Structures of size exactly a are created through nucleation at a rate k n . Additional monomer are added to the structure at the two ends with rate k g . For simplicity we assume that all the correct partners bind with the same rate k g . The master equation for X i , i + a −1 ( t ) is: Structures of size larger than critical size a and smaller than n grow by picking up monomers on either side, that is, for n −1 > j − i > a −1, Structures of size n are assumed to close up and form full rings, which are stable and inert.We numerically solved these equations in Mathematica with fixed values for different initial concentrations C i ( t = 0) and found the value of X ij ( t ) at large times when no further changes occur. We varied n between 25 and 50 with fixed a =10. Supplementary Note 3 contains numerical details. P-shaped structure . We carried out discrete-time stochastic simulations for nucleation and growth of the P-shaped structure, which is made of n =208 distinct square tiles; each tile has four distinct binding sites that bind only to their correct partners in Fig. 7(d) . We start the simulation with an integer c i ( t =0) copies of species i . At each discrete time step, we randomly choose to either nucleate a new seed of size a =18 or grow existing seeds. The probability of nucleating a seed S of critical size a =18 is where the product is over the a =18 species j ε S found in the seed S and λ N is a normalization constant. The probability of a pre-existing seed growing by picking up the correct tile of species i at a boundary site is . We reduce the numbers c i ( t + 1) = c i ( t ) − 1 for species i , which participate in nucleation or growth of seeds and run the simulation until no further nucleation or growth takes place (that is, tiles are fully depleted). The ratio of the constants λ N , λ G in the above probabilities of nucleation and growth is a free parameter that is not set by normalization and determines the relative speed of nucleation and growth processes. We report results for rapid nucleation (that is, a high ratio of λ N to λ G ), a limit in which depletion traps are severe. See Supplementary Note 3 for more details of the above Gillespie algorithm, including normalization and numeric details. Kinetic aggregation of colloids In our discrete-time stochastic simulations, we begin with a mixture of c A particles of type A and c B particles of type B such that c A , c B are positive integers with c A + c B = 1,000. Any structure composed of i A A and i B B particles is said to be of type i = ( i A , i B ). At each time step, we pick two random structures (including free particles), uniformly and without replacement, out of the mixture; let us say they are of type i = ( i A , i B ) and type j = ( j A , j B ). Then, we glue them together—producing a new structure of type k = ( i A + j A , i B + j B )—with a probability given by a kernel K ( i , j )ε[0,1] that depends on the mass and composition of the two structures. Hence, reactions (that is., gluing) between structures of type i and j happen at a rate c i c j K ( i , j ), where c i , c j are the numbers of the type i and j structures. The two original structures of type i and j are removed from the solution. Kernel K ( i , j ) implements the rule that A and B only bind to each other and not to themselves. Note that as an approximation, we track structures only by their overall composition (that is, numbers of A and B) and do not track the precise arrangement of the A, B particles within the structure. This approximation and corresponding details of the kernel K ( i , j ) are described in Supplementary Note 3 . We evolve the system in discrete time steps until no further gluing occurs, giving a final mix of structures that cannot react any further. How to cite this article: Murugan, A. et al . Undesired usage and the robust self-assembly of heterogeneous structures. Nat. Commun. 6:6203 doi: 10.1038/ncomms7203 (2015).